High-performance and site-directedin uteroelectroporation by a triple-electrode probe In utero electroporation is a powerful tool to transfect and manipulate neural-precursor cells of the rodent parietal cortex and their progeny in vivo . Although this technique can potentially target numerous brain areas, reliability of transfection in some brain regions is low or physical access is limited. Here we present a new in utero electroporation configuration based on the use of three electrodes, the relative position and polarities of which can be adjusted. The technique allows easy access and exceedingly reliable monolateral or bilateral transfection at brain locations that could only be sporadically targeted before. By improvement in the efficiency of the electrical field distribution, demonstrated here by a mathematical simulation, the multi-electrode configuration also extends the developmental timeframe for reliable in utero electroporation, allowing for the first time specific transfection of Purkinje cells in the rat cerebellum. In utero electroporation (IUE) is a simple and quick procedure to efficiently perform in vivo genetic manipulation of specific cell types at different brain locations [1] , [2] . This technique takes advantage of the fact that by targeting neural progenitors at the epithelium of the ventricular system, one can address specific populations of newborn neurons that will migrate to the various brain areas. Depending on the locations of the different progenitors in the neurogenic epithelia and on the embryonic stage, this results in a spatially and temporally restricted neuronal population carrying the gene of interest [1] , [2] , [3] , [4] , [5] , [6] , [7] . Transfection of neural progenitors of the brain area of interest is achieved by microinjection of plasmid DNA solution into the lumen of the ventricular system, followed by manually directing electrical pulses to the relevant neurogenic tissue. Current delivery is facilitated by extra-uterine forceps-type paddle electrodes, which contribute to physically holding the uterus and the yolk sac containing the embryo. The electric shocks destabilize the structure of the lipophilic cell membrane and induce the formation of transient electropores. Therefore, negatively charged DNA drifts towards the anode in the electric field, actively penetrating into the cell cytoplasm and allowing selective transfection of the neurogenic regions. With expertize, ~70–90% of born pups expresses the transfected plasmid appropriately [8] . Gene expression in neurons persists for a long time postnatally, and co-electroporation of fluorescent reporter genes enables visualization of targeted cells across development [5] , [7] . IUE was first described in 2001 by three independent reports as a means to achieve targeted gene expression in the developing parietal (somatosensory) cortex of the rodent in vivo [8] , [9] , [10] . Since then, owing to the simplicity and reliability of the procedure, the number of publications with IUE aiming at the somatosensory cortex has increased exponentially ( Supplementary Fig. S1 ). In parallel, as the first description, several investigators have developed IUE for gene targeting of other brain regions by tilting the extra-uterine paddle electrodes and orienting the position of the electric field along different axes [1] , [2] , [11] . In particular, specific electroporation of the hippocampus—first described in 2001 (ref. 8 ) and methodologically detailed in 2005 (ref. 12 ) and 2007 (ref. 13 )—was obtained by orienting the forceps-type electrode in the medio-lateral axes. Moreover, electroporation of the visual cortex was achieved in 2005 by orienting the forceps-type electrode along the antero-posterior axes [14] . However, notwithstanding the great scientific interest on both these brain regions, only two other articles for the hippocampus [12] , [13] and visual cortex [15] , [16] appeared in the first 6 years following their initial publications. Notably, in the same timeframe the number of publications on the somatosensory cortex raised to 35 ( Supplementary Fig. S1 ). This possibly indicates that reliability and consistency of IUE transfection was not straightforward for brain areas other than the somatosensory cortex. Indeed, although IUE has tremendous potentialities in targeting all cell populations in brain areas deriving from progenitors lining the walls of the ventricular system, the steric inaccessibility of embryos in utero to a tilted forceps-type electrode may have made it difficult or impossible to practically target theoretically attainable regions [6] , [17] . Here, we present an innovative IUE configuration that allows simple and highly consistent transfection at various brain locations. The method relies on the usage of three independent electrodes that upon an easy and highly reliable re-orientation of the electrode's positions and polarities results in a much improved accessibility to embryos in utero and a more efficient electric-field distribution, allowing a largely consistent expression of the genes of interest in the hippocampus, visual cortex, motor cortex and, for the first time to our knowledge, Purkinje cells in the cerebellum. Tripolar configuration for site-directed electroporation Given a good plasmid injection to reliably direct the DNA by the electric field across the various neurogenic brain regions, a key factor is an easy and consistent access of the extra-uterine electrodes to the embryos located in utero . To this aim, we adopted a combination of standard forceps-type electrodes and a third spare electrode, used to properly orient the electric field, positioned at 0° or 90°, with respect to the horizontal plane ( Fig. 1a ). Indeed, this configuration permitted both simple access to the rat embryos and reliable reproduction of the entire electroporation process, as the forceps-type electrode allowed holding the embryos in a reproducible manner, and the 0° or 90° angle was easily and consistently achieved with the third electrode (in contrast to the hard placing of the forceps-type electrode at 15–45° inclination previously described for targeted IUE of the hippocampus [13] ). Moreover, different brain regions could be targeted by simply reconfiguring the three electrode's polarities without changing their positions ( Fig. 1a ). 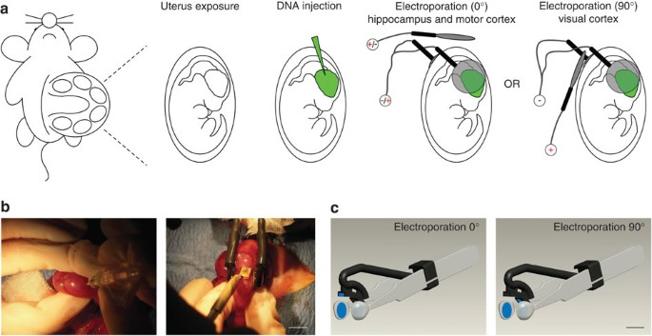Figure 1:Three-electrode configuration and device for improved IUE. (a) Schematic cartoon of the IUE procedure entailing DNA injection and electroporation by means of a standard forcipes-type electrode and a spare third electrode oriented at either 0 or 90°.(b) Representative pictures of the three-electrode configuration during surgery. (c) 3D model of the multi-electrode device. Scale bars, 10 mm. Figure 1b depicts the actual three-electrode configuration during a typical experiment. Figure 1: Three-electrode configuration and device for improved IUE. ( a ) Schematic cartoon of the IUE procedure entailing DNA injection and electroporation by means of a standard forcipes-type electrode and a spare third electrode oriented at either 0 or 90°. ( b ) Representative pictures of the three-electrode configuration during surgery. ( c ) 3D model of the multi-electrode device. Scale bars, 10 mm. Full size image Rat embryos at embryonic day (E) E17 were used to determine the optimal conditions for in vivo electroporation of the hippocampus and visual cortex. To visualize the transfected progenitor cells and their progeny at its final location, we injected in the ventricular system ( Fig. 1b , left) a plasmid carrying enhanced green fluorescent protein (EGFP; 1.5 μg μl −1 ) downstream of a strong and ubiquitous CAAG promoter. Injections for both areas were performed at the ipsilateral–lateral ventricle ( Fig. 2a , green regions; Supplementary Movies 1,2 ). Then, we applied square electric pulses (five pulses, amplitude 50 V, duration 50 ms and interval 150 ms) through the uterine wall to embryos, by physically holding them in parallel along the antero-posterior axis at the level of the lateral ventricle with the forceps-type electrodes ( Fig. 1a,b ). To finely address the electric field to the neurogenic epithelia ( Fig. 2a , asterisk), we placed the third electrode at 0° angle (hippocampus), or 90° (visual cortex), with respect to the horizontal plane ( Figs 1a,b and 2a ; Supplementary Movies 1,2 ). Finally, to orient the electric fields and direct the DNA, we simply varied the polarity of the electrodes. In particular, we connected the forceps-type electrodes to the positive pole (+) for transfection of the hippocampus, and to the negative pole (−) for transfection of the visual cortex ( Figs 1a and 2a ; Supplementary Movies 1,2 ). Consequently, the third electrode was connected to the negative pole in the first case and to the positive pole in the second one ( Figs 1a and 2a ; Supplementary Movies 1,2 ). EGFP-expressing cells were analysed in coronal sections at postnatal day (P) 2–21. Electroporation to the targeted areas resulted in confined areas of EGFP fluorescence, where a number of neurons had been generated and migrated ( Fig. 2b , Supplementary Figs S2, S3, S4 ). In our experimental conditions, we obtained easy, highly efficient and reliable electroporation of the targeted areas ( Fig. 2b ). In particular, we successfully transfected 90.1±2.0% of live pups for the hippocampus ( n= 119) and 91.7±4.6% for the visual cortex ( n= 39, Table 1 ). Then, we tested the versatility of the three-electrode configuration for specific targeting of the motor cortex. This brain region has been only recently targeted [18] , [19] with the standard bipolar electrode, possibly because it requires a 90° tilting of the forceps-like electrode along the medio-lateral axes, hardly achievable considering the position of the embryos in the uterus. As for the hippocampus, we performed injections at the ipsilateral–lateral ventricle ( Fig. 2a , green region; Supplementary Movie 3 ) and applied square electric pulses by forceps-type electrodes at the level of the lateral ventricle and by the third electrode at 0° angle with respect to the horizontal plane. Conversely, to target the motor cortex, we connected the standard electrodes to the negative pole and the third electrode to the positive pole ( Figs 1a and 2a ; Supplementary Movie 3 ). In this condition, we successfully transfected 91.4±4.4% ( n= 37) of live pups ( Fig. 2b , Supplementary Fig. S5 ), perfectly in line with the hippocampus and visual cortex ( Table 1 ). Finally, in agreement with what has been previously found in the somatosensory cortex with the standard bipolar configuration [20] , for each brain area transfected by the three-electrode configuration, we exclusively targeted pyramidal (excitatory) neurons, as confirmed by immunohistochemistry for calcium calmodulin kinase II and γ-aminobutyric acid, specific markers of excitatory and inhibitory cells, respectively ( Supplementary Fig. S6 ). 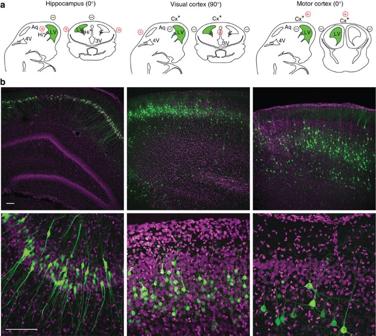Figure 2:Site-directedIUEof different brain areas. (a) Schematic representation of the relationship among the location of neural progenitors (*), injection site (green) and the relative position of the electrodes (red, positive pole; black, negative pole) to target different brain areas. LV: lateral ventricle, 4v: fourth ventricle. (b) Confocal images at low (top) and high (bottom) magnifications of representative fields from coronal hippocampal (left), visual cortical (middle) and motor cortical slices (right) with electroporated cells (green). 3v: third ventricle. Sections were counterstained with Hoechst (magenta). Scale bars, 100 μm. Figure 2: Site-directed IUE of different brain areas. ( a ) Schematic representation of the relationship among the location of neural progenitors (*), injection site (green) and the relative position of the electrodes (red, positive pole; black, negative pole) to target different brain areas. LV: lateral ventricle, 4v: fourth ventricle. ( b ) Confocal images at low (top) and high (bottom) magnifications of representative fields from coronal hippocampal (left), visual cortical (middle) and motor cortical slices (right) with electroporated cells (green). 3v: third ventricle. Sections were counterstained with Hoechst (magenta). Scale bars, 100 μm. Full size image Table 1 Three-electrode configuration allows high-performance in utero electroporation at different brain regions and embryonic stages. Full size table Tripolar configuration allows bilateral transfection In cases when we filled both ventricles with DNA by a monolateral injection plus few minutes waiting time for diffusion in the contralateral ventricle ( Fig. 3a ), a single electroporation episode could nicely transfect both hemispheres in a symmetric fashion for the hippocampus, visual cortex and motor cortex ( Fig. 3b ; Supplementary Fig. S7 ). This is a remarkable feature of the new electroporation configuration as (i) for the hippocampus, visual cortex and motor cortex, which have low transfection efficiency per se with standard IUE, would be very challenging, and possibly not feasible, to electroporate both hemispheres in the same animal by the two independent episodes of electroporation required by standard IUE; (ii) bilateral electroporation with the standard configuration in easily transfectable regions like the already described prefrontal cortex [11] or the somatosensory cortex (tested here for direct comparison) still requires two independent episodes of electroporation, which although inducing transfection in both hemispheres, hardly achieve good degree of symmetry of EGFP cell location [11] ( Fig. 3c , arrow), inevitably resulting in undesired transfection of areas different from the original target (for example, contralateral cingulate cortex; Fig. 3c , arrowheads). 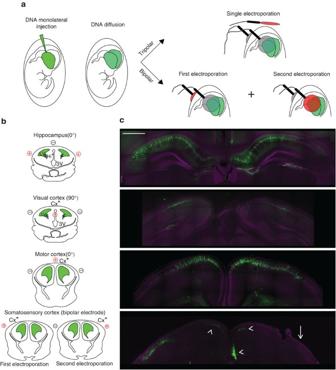Figure 3:Bilateral transfection of both hemispheres with a single electroporation episode. (a) Schematic representation of bilateralin uterotransfection entailing monolateral injection in one ventricle, filling of the contralateral ventricle by diffusion, and electroporation by a single episode (three-electrode configuration) or two consecutive episodes (two-electrode configuration) for bilateral transfection of different brain areas. Grey and red electrodes represent opposite polarities. (b) Schematic representation of the relationship among the location of neural progenitors (*), injection site (green) and the relative position of the electrodes (red, positive pole; black, negative pole) to target different brain areas. LV: lateral ventricle. 3v: third ventricle. (c) Representative confocal images of bilateral and symmetrical distribution of EGFP-transfected cells (green) obtained by single electroporation with the three-electrode configuration in the hippocampus, visual cortex and motor cortex. Bilateral electroporation in the somatosensory cortex was performed as the only possible reliable comparison by the two-electrode configuration. Good symmetric distribution of EGFP cell location was hardly achieved (arrow) with the two independent electroporation episodes, and predicted undesired electroporation of the cingulate cortex was also present (arrowheads). Sections were counterstained with Hoechst (magenta). Scale bars, 500 μm. Figure 3: Bilateral transfection of both hemispheres with a single electroporation episode. ( a ) Schematic representation of bilateral in utero transfection entailing monolateral injection in one ventricle, filling of the contralateral ventricle by diffusion, and electroporation by a single episode (three-electrode configuration) or two consecutive episodes (two-electrode configuration) for bilateral transfection of different brain areas. Grey and red electrodes represent opposite polarities. ( b ) Schematic representation of the relationship among the location of neural progenitors (*), injection site (green) and the relative position of the electrodes (red, positive pole; black, negative pole) to target different brain areas. LV: lateral ventricle. 3v: third ventricle. ( c ) Representative confocal images of bilateral and symmetrical distribution of EGFP-transfected cells (green) obtained by single electroporation with the three-electrode configuration in the hippocampus, visual cortex and motor cortex. Bilateral electroporation in the somatosensory cortex was performed as the only possible reliable comparison by the two-electrode configuration. Good symmetric distribution of EGFP cell location was hardly achieved (arrow) with the two independent electroporation episodes, and predicted undesired electroporation of the cingulate cortex was also present (arrowheads). Sections were counterstained with Hoechst (magenta). Scale bars, 500 μm. Full size image Electroporated neurons are viable Next, to assess the viability of transfected cells, we performed whole-cell patch-clamp recordings in acute visual cortical slices (P11–13) from wild-type neurons and neurons transfected in utero (by the triple-electrode configuration) with EGFP to measure basic membrane properties (membrane resistance, membrane capacitance and membrane resting potential), neuronal output properties (action potential firing) and extent of synaptic integration (spontaneous postsynaptic currents; Fig. 4 , Supplementary Table S1 ). We found that EGFP-transfected cells did not show any significant difference compared with controls. Altogether, these data demonstrate that our new three-electrode configuration and device permit to drastically increase the efficiency of transfection in brain areas other than the somatosensory cortex, still preserving neuron viability, single neuronal-population target selectivity, and easiness and rapidity of procedure, all key to the success of standard IUE [5] . 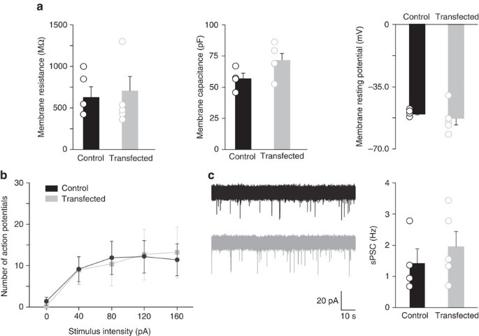Figure 4:Electrophysiological properties of transfected neurons. (a) Basic membrane properties of layer II/III visual cortical neurons transfected (E17.5) with EGFP (n=5) by the three-electrode configuration in comparison with control wild-type (WT) cells (n=4). Patch-clamp recordings were performed at P11-13. Membrane resistance, membrane capacitance and membrane resting potential did not show any significant difference (Student'st-test,P>0.05). (b) The same set of EGFP-transfected and control cells did not show statistically significant difference in spike discharge (Student'st-test,P>0.05). (c) Spontaneous postsynaptic currents (sPSC; example traces on the left; control WT, black; EGFP-transfected, grey) were also comparable in both conditions (Student'st-test,P>0.05). All histograms represent average±s.e.m., and hollow circles represent each recorded cell. Figure 4: Electrophysiological properties of transfected neurons. ( a ) Basic membrane properties of layer II/III visual cortical neurons transfected (E17.5) with EGFP ( n =5) by the three-electrode configuration in comparison with control wild-type (WT) cells ( n =4). Patch-clamp recordings were performed at P11-13. Membrane resistance, membrane capacitance and membrane resting potential did not show any significant difference (Student's t -test, P >0.05). ( b ) The same set of EGFP-transfected and control cells did not show statistically significant difference in spike discharge (Student's t -test, P >0.05). ( c ) Spontaneous postsynaptic currents (sPSC; example traces on the left; control WT, black; EGFP-transfected, grey) were also comparable in both conditions (Student's t -test, P >0.05). All histograms represent average±s.e.m., and hollow circles represent each recorded cell. Full size image Efficiency of tripolar electroporation configuration To directly compare the reliability of our new technique to standard IUE, we performed parallel electroporations with the tripolar and bipolar configurations for the hippocampus, visual cortex and motor cortex with the same operator and under the same experimental conditions. Indeed, no data had been reported on the efficiency of standard IUE transfection in these brain regions, and the low number of publications reporting IUE of the hippocampus and visual cortex is only an indirect evidence of possible technical issues. We found an efficiency of transfection of 18.7±6.2% ( n =42), 51.8±5.8% ( n =37) and 36.4±9% ( n =33) for the hippocampus, visual cortex and motor cortex, respectively. This is significantly much lower than the respective 90.1±2.0% ( n =119), 91.7±4.6% ( n =39) and 91.4±4.4% ( n =37) obtained with the three-electrode configuration ( Table 1 ). On the other end, survival rate of embryos electroporated with the tripolar configuration did not differ from that of the standard configuration (tripolar configuration: 71.4±5.1, n =161, 14 litters; bipolar configuration: 70.8±5.8, n =154, 15 litters). Then, to optimize the new IUE configuration, we realized and tested an electrode device allowing even easier handling and more rapid positioning of the electrodes ( Fig. 1c , Supplementary Movies 1,2,3 ). In particular, we designed the device to give full control and maximum reproducibility into the spatial configuration of the electrodes to the operator with one hand, and to have the other hand free to manipulate the embryos. Electric-field intensity of tripolar configuration As the ~90% reliability of transfection with our three-electrode configuration for the hippocampus, visual cortex and motor cortex appeared slightly higher than the reported transfection efficiency achieved by other laboratories for the somatosensory cortex with the bipolar electrode [8] (in our case, 80.6±4.4%, n =140; Table 1 ), we challenged our IUE configuration on this yield issue. We performed electroporation with the two-electrode and three-electrode probes (to target the highly reliable somatosensory cortex and motor cortex, respectively) at a lower voltage (20 V), previously reported to decrease the efficiency of transfection in standard IUE [8] . Interestingly, by delivering 20-V pulses, we transfected an expected [8] 30.1±7.8% ( n= 29) only of live pups with the standard electrode configuration in comparison with the high 68.6±11.3% ( n= 16) obtained with the three-electrode configuration ( Table 1 ). To better understand this experimental evidence, we performed a modelling study on the spatial distributions of the electric field induced by the potential applied to the electrodes (for the tripolar and for the bipolar probes) within a three-dimensional (3D) reconstruction of the embryo's brain at E16. We took into account the geometry [21] of the embryonic brain, the permittivity and conductivity [22] , [23] of the brain tissue and that of the surrounding and ventricle media [21] , [22] along with the relative electrode positions and voltages applied (50 V). X–Y sections obtained from the simulations for the hippocampus and motor cortex clearly showed that in the three-electrode configuration the electric field was indeed directed towards the different neurogenic regions (asterisk in Fig. 5a ; Fig. 5a,b ). Moreover, the electric field appeared symmetrical, supporting the transfection of both brain hemispheres in experimental animals loaded in both ventricles. Of note, the simulation of the electric field for the transfection of the somatosensory cortex with the standard configuration also supported the experimental evidence of undesired transfection of the cingulate cortex in the case of DNA loading of both ventricles (white # in Fig. 5b ). Along with the directionality and symmetry, the introduction of the third electrode positioned at 0° resulted in highly localized and extremely effective (in terms of field intensity) stimulation of the various neurogenic regions in comparison with the standard configuration ( Fig. 5b ). This possibly resulted from the distance between the cathode and anode, which is much smaller than in the case of bipolar electrodes. Altogether, these results supported the high efficiency of transfection in brains experimentally electroporated by our three-electrode configuration at low voltages, and also opened the experimental perspective towards a really promising scenario. 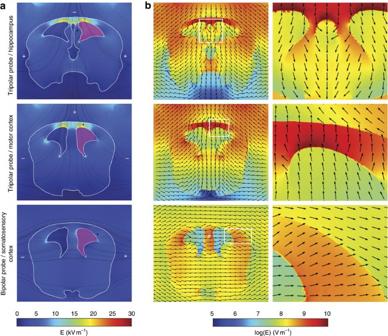Figure 5:Simulation of electric-field distributions highlights the high intensity obtained with the triple-electrode probe. (a) Coronal views of the electric-field intensity (in linear scale) for the three-electrode probe in comparison with the standard bipolar configuration. Stream lines for the electric field are indicated in black. Minus and plus indicate the actual position and polarity of the electrodes. Magenta indicates the site of injection of the DNA. Asterisks indicate the diverse neurogenic regions. (b) Images at low (left) and high magnification from boxed regions (right), showing electric-field intensity (in logarithmic scale) along with field direction (black arrows) pointing to the diverse neurogenic areas indicated by the asterisk ina. # indicates the neurogenic region of neurons of the cingulate cortex. All images are color-coded according to the pseudo-color scales at the bottom. Figure 5: Simulation of electric-field distributions highlights the high intensity obtained with the triple-electrode probe. ( a ) Coronal views of the electric-field intensity (in linear scale) for the three-electrode probe in comparison with the standard bipolar configuration. Stream lines for the electric field are indicated in black. Minus and plus indicate the actual position and polarity of the electrodes. Magenta indicates the site of injection of the DNA. Asterisks indicate the diverse neurogenic regions. ( b ) Images at low (left) and high magnification from boxed regions (right), showing electric-field intensity (in logarithmic scale) along with field direction (black arrows) pointing to the diverse neurogenic areas indicated by the asterisk in a . # indicates the neurogenic region of neurons of the cingulate cortex. All images are color-coded according to the pseudo-color scales at the bottom. Full size image Tripolar configuration for transfection of Purkinje cells IUE selectivity for diverse brain areas has been recognized to depend on the specific neurogenic region targeted during the prenatal stages, but also on the proper selection of the time for electroporation. For example, in the somatosensory cortex, targeting progenitor cells in the ventricular zone at early stages results in the transfection of cells that mainly differentiate into pyramidal neurons of cortical layer VI/V and IV, whereas electroporation at later stages results in transfection of layer II/III neurons [1] , [11] . This reflects the pattern of cortical development, whereby early born neurons migrate to deep layers of the cortex and later born neurons migrate to superficial layers [24] . However, electroporation of younger animals is challenging. Indeed, survival of electroporated embryos drastically decreases with age [8] , owing to fact that the electroporation electrodes rest closer to the embryo's heart, affecting its rhythm with the strong electric pulses [5] . Therefore, the impossibility to target some brain regions [6] , [17] may depend on both the physical accessibility of the embryos to the forceps-type electrodes and the low survival rate of the embryos with electroporation at young ages. One example are neurons in the cerebellum (granule and Purkinje cells), which originate at the level of the roof of the fourth ventricle [25] . Thus, IUE would require a 90° tilting of the bipolar electrode along the medio-lateral axes, hardly achievable when embryos are located in the yolk sack and utero . Indeed, electroporation of the cerebellum was first performed postnatally, when one can easily access the pup from all angles [26] . However, electroporation of pups only targeted the granule cell neurons, as they are generated postnatally. Conversely, Purkinje cells are generated at early embryonic stages, and have never been targeted before, possibly because of the combined difficulty of accessing the roof of fourth ventricle with the standard bipolar electrode in utero together with the low survival rate of embryos electroporated at early stages. Our new IUE configuration was tested to this aim, as it easily directed the electric field to 90° angle and it allowed efficient electroporations at lower voltages to increase the survival rate of embryos at early stages. We injected rat embryos at E14.5–15.5 in the fourth ventricle ( Fig. 6a , green region; Supplementary Movie 4 ), and we applied low (35 V) voltage pulses (duration 50 ms and interval 150 ms). To address the electric field to the neurogenic epithelium ( Fig. 6b , asterisk), we placed the forceps-type electrode at the level of the fourth ventricle and placed the third electrode at 90° with respect to the horizontal plane. The forceps-type electrodes were connected to the negative pole and the third electrode to the positive pole ( Fig. 6b ; Supplementary Movie 4 ). EGFP-expressing cells were analysed in sagittal sections at P14–21 ( Fig. 6c and Supplementary Fig. S8 ). Strikingly, in the cerebellum we exclusively transfected Purkinje cells ( Supplementary Fig. S9 ), which were numerous when electroporation was performed at E14.5, whereas they were isolated upon IUE at E15 ( Fig. 7 ), allowing their precise morphological reconstructions ( Supplementary Movie 5 ). Notably, in utero transfection performed only half a day later (E15.5) resulted in exclusive transfection of giant buttons at mossy fibres, in line with the narrow window for Purkinje cell-type development [25] . Electroporation efficiency was reliable, and success rate attested around 57.7±7.7% of live pups ( n =41; Table 1 ). We note that although the success rate was lower than what we obtained for the other brain regions, it may simply result from the more challenging injection conditions, independently of our three-electrode-based targeting method. Indeed, electroporation for the hippocampus, visual cortex and motor cortex were performed at E17, whereas electroporation for the cerebellum was performed at E14.5–15.5, when embryos are considerably smaller in size. Altogether, these results demonstrate that our new IUE configuration, by assuring higher accessibility to embryos in utero and lower electroporation voltages, allows easy and reliable targeting of cells at early embryonic stages and consequent in utero transfection of cell types and brain areas never attained before. 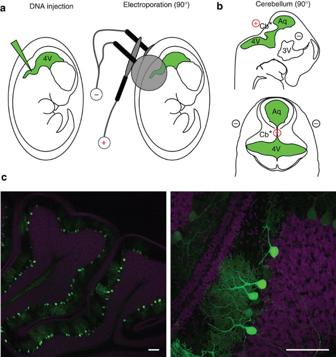Figure 6: IUEof cerebellar Purkinje cells. (a) Schematic cartoon of the IUE procedure entailing DNA injection in the fourth ventricle, and electroporation by means of a triple-electrode configuration for cerebellum. 4V: fourth ventricle, Aq: aqueous. (b) Schematic representation of the relationship among the location of neural progenitors (*), injection site (green) and the relative position of the electrodes (red, positive pole; black, negative pole) to target Purkinje cells. (c) Confocal images at low (left) and high (right) magnifications of representative fields from sagittal slices of cerebellum with electroporated cells (green). Sections were counterstained with Hoechst (magenta). Scale bars, 100 μm. Figure 6: IUE of cerebellar Purkinje cells. ( a ) Schematic cartoon of the IUE procedure entailing DNA injection in the fourth ventricle, and electroporation by means of a triple-electrode configuration for cerebellum. 4V: fourth ventricle, Aq: aqueous. ( b ) Schematic representation of the relationship among the location of neural progenitors (*), injection site (green) and the relative position of the electrodes (red, positive pole; black, negative pole) to target Purkinje cells. ( c ) Confocal images at low (left) and high (right) magnifications of representative fields from sagittal slices of cerebellum with electroporated cells (green). Sections were counterstained with Hoechst (magenta). Scale bars, 100 μm. 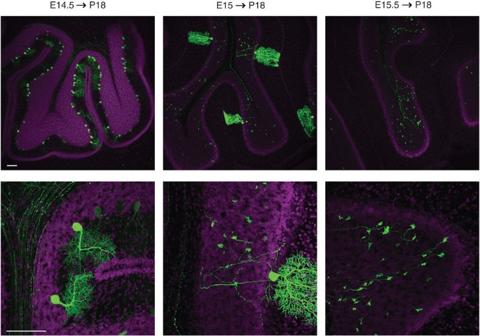Figure 7:A narrow time window exists for Purkinje cell transfection. Effective transfection of Purkinje cells was achieved by electroporation at E14.5. Electroporation performed at E15 resulted in sparse Purkinje cell transfection, whereas half a day later (E15.5) only giant buttons at mossy fibres were found EGFP positive (green). Upper and lower images were acquired with X10 and X40 magnification, respectively. Sections were counterstained with Hoechst (magenta). Scale bars, 100 μm. Full size image Figure 7: A narrow time window exists for Purkinje cell transfection. Effective transfection of Purkinje cells was achieved by electroporation at E14.5. Electroporation performed at E15 resulted in sparse Purkinje cell transfection, whereas half a day later (E15.5) only giant buttons at mossy fibres were found EGFP positive (green). Upper and lower images were acquired with X10 and X40 magnification, respectively. Sections were counterstained with Hoechst (magenta). Scale bars, 100 μm. Full size image We described a new IUE configuration and device based on the use of three electrodes that allowed easy and reliable transfection at brain locations other than the somatosensory cortex, including Purkinje cells of the cerebellum, which has never been reported before. Upon DNA loading of both ventricles, this configuration induced bilateral transfection in both brain hemispheres by a single electroporation episode. Moreover, at lower voltages, the new three-electrode configuration allowed higher efficiency of transfection than the conventional bipolar one. Finally, we developed a 3D model for the computation of the spatial distributions of the electric field induced by the voltages applied to the electrodes within the brain that accounted for the versatility, high reliability and high efficiency of the new IUE configuration. The importance of our new configuration in comparison with other methods arises in those applications where tissue and circuit integrity are essential points, and in those where traditional IUE is the limiting step of the experimental approach. In the recent past, IUE has been indeed the method of choice for rapid gain and loss-of-function studies in the embryonic cerebral cortex [1] . The success of IUE is demonstrated by the increasing number of research articles taking advantage of this technique and by the numerous (ten) reviews [1] , [2] , [3] , [4] , [6] , [11] , [27] , [28] , [29] , [30] on this methodology published in the last 10 years. This success mostly depends on the simplicity, quickness and reliability of the technique [5] . Another very interesting feature of IUE is that it has the potential to target all brain areas, although results obtained so far may indicate that its extreme versatility is to the detriment of reliability. For example, we described that a total of only two publications each reported electroporation of the hippocampus and visual cortex in the first 6 years after their initial description. On the other hand, the low number of publications could also simply depend on the bias of the extensive usage of IUE in the research field of development (migration, proliferation and differentiation) for which the parietal cortex is broadly used as a model, rather than the hippocampus or visual cortex, which are good models for plasticity, physiological or behavioural studies. However, there are instances when, for example, the hippocampus is the system of choice also for investigation on neuronal development. Indeed, in the field of axonal polarization, hippocampal cells in culture have been used for more than 20 years [31] . As IUE has arisen as an incredibly powerful technique to study neuronal development, numerous independent laboratories in the polarity field have also turned to this in vivo system to back up their in vitro data [32] , [33] , [34] , [35] , [36] , [37] , [38] , [39] . However, the anomaly rests in the fact that whether in all but one [39] of these studies hippocampal cultures remained the in vitro system of choice, in vivo data were obtained in somatosensory cortex neurons targeted with the IUE, which may again indicate technical issues in reliably targeting the hippocampus. Surprisingly, although two specific method articles already described in full the electroporation of the hippocampus [12] , [13] , no quantitative data on the efficiency of electroporation of the hippocampus and visual cortex had been available. For the first time, we directly provided quantitative data on the efficiency of electroporation of the hippocampus and visual cortex with the standard bipolar electrode and found it overwhelmingly lower than what attained in the parietal cortex [8] . Our new three-electrode probe completely filled the gap in the electroporation efficiency of the different brain areas. Certainly, we cannot exclude that particularly skilled operators with extensive and long-lasting training may achieve better efficiency for the hippocampus, visual cortex and motor cortex also with the standard bipolar electrode. However, this would be in sharp contrast with the key features of IUE that entails simplicity and rapidity [5] . Finally, even though Purkinje cells are one of the systems of choice to study dendrite growth and synapse elimination during development [40] , [41] , IUE has never targeted this cell population. This possibly derived from the fact that electroporation of Purkinje cells would require risky electroporation at early embryonic stages together with electroporation at the upper fourth ventricle, difficult to access with the standard bipolar configuration. Here, we consistently transfected Purkinje cells of the cerebellum by our new IUE configuration. Indeed, our system allowed reliable electrode access to the upper fourth ventricle and it enabled the use of lower voltages for comparable transfection outcomes, and therefore it proved to be well suited for electroporation of younger embryos. Thus, the new IUE configuration by an extremely easy-to-realize technical improvement allowed to overcoming the most severe limitations of standard IUE. Possibly, this will be profoundly influential for future developmental studies in areas other than the parietal cortex. The introduction of a third electrode to gain better access to different neurogenic areas is a conceptual advance in IUE technique. The system proved versatile as just by switching the polarities of the electrodes we could target both the hippocampus and motor cortex. In the near future, new application by varying the number together with the polarities of the electrodes may allow transfection of other brain areas never targeted before. To this aim, the mathematical 3D simulation of the electric field—which we introduced here for the first time to support the versatility, high reliability and efficiency of the new three-electrode configuration—should be considered as an important add-on to the IUE protocol, and may constitute a future predictive tool for the optimization of new transfection protocols. Moreover, the 3D simulation also showed that the electric field is bilateral and mostly symmetric in the case of the three-electrode configuration. This is an extremely interesting feature, taken into account the increasing interest of IUE-transfected animals for behavioural studies [11] , [28] . Indeed in these kinds of experiments, filling of both ventricles with DNA followed by two successive electroporations with the standard bipolar electrode is usually performed in order to achieve the indispensable bilateral and possibly symmetric transfection. The bilateral and symmetric field that we generated with our new configuration allowed to reliably transfect both hemispheres with a single episode of current delivery, halving the risk of embryonic death [5] . Moreover, the bilateral electroporation with the standard configuration inevitably generated undesired transfection of the cingulate cortex in both hemispheres. This may be partially (just for one hemisphere) avoided only by filling one ventricle at a time [11] , requiring, nevertheless, two independent injections harmful for brain damage. Finally, in the last 5 years IUE has acquired increasing importance owing to its coupling to other useful techniques such as RNA interference and in vivo imaging. In particular, tamoxifen-inducible Cre-ER(T) recombinase system [42] and optogenetics [43] coupled to our reliable new IUE configuration will allow consistent, temporally restricted and subtle modulation of neuronal activity in brain areas extensively studied for neuronal plasticity (hippocampus and visual cortex), making also this experimental field easily accessible to the most. Moreover, besides DNA, any charged macromolecules, such as dyes, chemical reagents and antibodies, can be targeted by IUE [3] , [6] , [29] to tissues other than the nervous system, including somites, limb derm and cardiac tissue [4] . In this light, the new high-performance and site-directed IUE represents a conceptual advance to IUE technique, and will possibly become a new research tool opening avenues for experimental investigation of novel fundamental biological questions in the near future. DNA vectors The complementary DNA sequence encoding for the fluorescent protein EGFP or Td-Tomato was inserted into the pCAAG-IRES expression vector bearing a modified chicken β-actin promoter with a cytomegalovirus immediate early enhancer, which conferred high and long-lasting expression in vivo [44] . In utero electroporation Animal care and experimental procedures were conducted in accordance with the Italian Institute of Technology licensing and the Italian Ministry of Health. The day of mating (limited to 4 h in the morning) was defined as embryonic day zero (E0), and the day of birth was defined as postnatal day zero (P0). E14.5–15.5 (cerebellum) or E17 (hippocampus and cortex) timed-pregnant Sprague Dawley rats (Harlan Italy SrL, Correzzana, Italy) were anesthetized with isoflurane (induction, 3.5%; surgery, 2.5%), and the uterine horns were exposed by laparotomy. The DNA (1–2 μg μl −1 in water) together with the dye Fast Green (0.3 mg ml −1 ; Sigma, St Louis, MO, USA) was injected (5–6 μl) through the uterine wall into one of the lateral ventricles (hippocampus and cortex) or the fourth ventricle (cerebellum) of each embryos by a 30-gauge needle (Pic indolor, Grandate, Italy). After soaking the uterine horn with a phosphate-buffered saline (PBS) solution, the embryo's head was carefully held between tweezer-type circular electrodes (hippocampus, visual cortex and motor cortex: 10 mm diameter; cerebellum: 5 mm diameter, Nepa Gene, Chiba, Japan), while the third electrode (7×6×1 mm, gold-plated copper) was accurately positioned at different locations, as described in Fig. 1 . For the electroporation, five electrical pulses (hippocampus and cortex: amplitude, 50 V; duration, 50 ms; intervals, 150 ms; cerebellum: amplitude, 35 V; duration, 50 ms; intervals, 150 ms) were delivered with a square-wave electroporation generator (CUY21EDIT, Nepa Gene; ECM 830, BTX, Harvard Apparatus). In a subset of experiments, electroporation of somatosensory and motor cortices were performed at 20 V. For bilateral electroporation experiments, DNA filling in both ventricles was achieved by a single monolateral injection (plus few minutes waiting time for diffusion in the contralateral ventricle) to avoid excessive brain damage. For all animals, the uterine horns were returned into the abdominal cavity after electroporation, and embryos allowed continuing their normal development. For surgery on E14.5–15.5 embryos, illumination was performed with a flexible optic fibre with a cold light source (Olympus KL1550 LCD) from behind the embryo, whereas for surgery on E17 embryos illumination was achieved by two rigid fibres placed above the operating table. In some experiments, a plasmid encoding a red fluorescent protein (Td-Tomato; 1.5 μg μl −1 ) was injected as reporter. Slice histology and immunostaining P2–21 brains were fixed by transcardial perfusion of 4% paraformaldehyde in PBS. Brains were sectioned coronally (hippocampus, visual cortex and motor cortex) or sagittally (cerebellum) at 80 μm thickness with a vibratome (model 1000plus; Vibratome, St Louis, MO, USA). Free-floating slices were permeabilized and blocked with PBS containing 0.3% Triton X-100, 10% normal goat serum (NGS) and 0.2% bovine serum albumin (BSA). Primary antibodies were incubated in PBS containing 0.3% Triton X-100, 5% NGS and 0.1% BSA (rabbit anti-GABA, 1:1000 (Sigma); mouse anti-CaMKII, 1:100 (Thermo Scientific, San Jose, CA, USA); mouse anti-calbindin, 1:100 (Sigma)). Immunostaining was detected using Alexa 488, Alexa 546 or Alexa 647 fluorescent secondary antibody 1:1000, (Invitrogen, San Giuliano Milanese, Italy), incubated in PBS containing 0.3% Triton X-100, 5% NGS and 0.1% BSA. Slices were counterstained with Hoechst (50 μg μl −1 ; Sigma), mounted in ProLong Gold Antifade Reagent (Invitrogen) and examined with confocal microscopy. Confocal image acquisition For analysis of electroporated brain areas, low-magnification images were acquired on a confocal laser-scanning microscope (TCS SP5; Leica Microsystems, Milan, Italy) using a X10 oil immersion objective (numerical aperture (NA) 0.3). Volume z-stacks (80 μm thick) for each experimental condition were acquired, and the Z -series images were collapsed with a maximum intensity projection to a 2D representation. In the same manner, high-magnification images were acquired with a X40 oil immersion objective (NA 1.3), and post processed to extract the details of the cellular morphology and to obtain the 3D cell reconstruction. Images with larger fields of view attesting the performances of the bilateral electroporation were acquired with a NeuroLucida workstation (MicroBrightField, Magdeburg, Germany) equipped with a X10 air objective (NA 0.3). Electric-field simulation A full 3D volumetric model of the rat brain (developmental stage E16) was reconstructed starting from serial coronal sections imported from the rat brain atlas [21] , taking care of the correct definition of the regions of interest corresponding to the ventricles within the brain boundaries. The platform COMSOL multiphysics (COMSOL SrL, Brescia, Italy) was adopted to build the mesh structure for the complete volume including the ventricles, the brain, the medium around it and the electrodes for the electroporation. In order to define the correct electrical configuration of the system, distinct permittivity and conductivity values were recovered from the data available in literature into the 10–100-Hz frequency band [22] , [23] for the different electrical domains. The position of the electrodes for the different experimental configurations as well as their proper polarities were set as boundary conditions at the beginning of the simulation runs. The steady-state configuration of the system was computed, and the electric-field intensity and orientation maps were generated for the whole brain after reaching the convergence. Electrophysiology All functional analyses were performed in P11–13 animals that had been previously electroporated in utero (E17.5) with the pCAAG-EGFP construct, as described above. 400-μm coronal slices of the visual cortex were acutely isolated with a vibratome (VT1000S, Leica Microsystems) in ice-cooled cutting solution with the following composition (in mM): 0.1 MgCl 2 ; 2.5 KCl; 1.25 NaH 2 PO 4 ; 2 MgSO 4 ; 0.1 CaCl 2 ; 26 NaHCO 3 ; 206 Sucrose and 12 D -Glucose (~300 mOsm, pH 7.4), oxygenated with 95% O 2 and 5% CO 2 . The slices were incubated at 35 °C in artificial cerebral spinal fluid with the following composition (in mM): 124 NaCl; 2.5 KCl; 1.25 NaH 2 PO 4 ; 2 MgSO 4 ; 2 CaCl 2 ; 26 NaHCO 3 and 12 D -Glucose (~310 mOsm, pH 7.4), oxygenated with 95% O 2 and 5% CO 2 . After 1 h recovery, slices were transferred to a recording chamber at room temperature and perfused with artificial cerebral spinal fluid at a rate of 1.5 ml min −1 . Whole-cell patch-clamp recordings were made from layer II/III neurons of the visual cortex. Neurons derived from electroporated progenitor cells were identified by EGFP fluorescence using an upright fluorescence microscope (BX51 WI; Olympus, Italy). Glass micropipettes (resistance, 4–8 MΩ) were filled with an internal solution of (in mM): 120 K-Gluconate; 20 KCl; 10 HEPES; 0.1 EGTA; 2 MgCl 2 ; 10 phosphocreatine Na 2 ; 2 Mg 2 + ; 0.25 Na 2 GTP (~300 mOsm, pH 7.4). The membrane resting potential was measured immediately after whole-cell access at zero current. To elicit spike discharge, a depolarizing current pulse was delivered (+40 pA, 500 ms, five steps) using Clampex 10.2 software (Molecular Devices, Sunnyvale, CA, USA). For spontaneous postsynaptic currents, the holding potential was set at −70 mV and gap-free recordings were performed for 5 min. Data were analysed off-line with Clampfit software (Molecular Devices). Criteria for accepting a recording included an input resistance >200 MΩ, and a series resistance <50 MΩ. Capacitance, input and series resistance were measured online with Clampex 10.2. All recordings were performed at room temperature with a Multiclamp 700B amplifier (Molecular Devices). Data were sampled at 20 KHz and filtered at 5 KHz. How to cite this article: dal Maschio, M. et al . High-performance and site-directed in utero electroporation by a triple-electrode probe. Nat. Commun. 3:960 doi: 10.1038/ncomms1961 (2012).